Atomic scale study of the life cycle of a dislocation in graphene from birth to annihilation Dislocations, one of the key entities in materials science, govern the properties of any crystalline material. Thus, understanding their life cycle, from creation to annihilation via motion and interaction with other dislocations, point defects and surfaces, is of fundamental importance. Unfortunately, atomic-scale investigations of dislocation evolution in a bulk object are well beyond the spatial and temporal resolution limits of current characterization techniques. Here we overcome the experimental limits by investigating the two-dimensional graphene in an aberration-corrected transmission electron microscope, exploiting the impinging energetic electrons both to image and stimulate atomic-scale morphological changes in the material. The resulting transformations are followed in situ , atom-by-atom, showing the full life cycle of a dislocation from birth to annihilation. Our experiments, combined with atomistic simulations, reveal the evolution of dislocations in two-dimensional systems to be governed by markedly long-ranging out-of-plane buckling. The central role of dislocations in determining the behavior of solid-state matter has been extensively investigated in materials sciences since the first formulation of the dislocation concept at the beginning of the twentieth century [1] , [2] , [3] and their experimental discovery 50 years later [4] . However, up until now, atomic-scale studies of creation, migration and annihilation of dislocations have been reserved for theory and atomistic simulations, as monitoring changes in the structure of materials with atomic resolution has been well beyond the spatial and temporal limits of experimental characterization techniques. Lower-resolution observations of dislocation motion have been made already in the 50’s (ref. 5 ), using a transmission electron microscope (TEM). TEM has proven to be a powerful tool for studying the structure and arrangement of dislocations, with seminal work laid out by Cockayne et al . [6] in 1969 by the introduction of the weak beam method [6] , [7] . Recently, Hashimoto et al . [8] showed the appearance of a dislocation in sp 2 -hybridized carbon, and Warner et al . [9] presented atomically resolved aberration-corrected high-resolution TEM (AC-HRTEM) images of dislocations in graphene, demonstrating the basic glide and climb steps. In both works, the appearance of the dislocations was attributed to displacement and reorganization of carbon atoms. However, the actual steps in the underlying dynamical process have not yet been observed experimentally at the atomic scale. This is what we report here—thanks to the two-dimensional (2D) nature of graphene, which facilitates AC-HRTEM observations of the structural changes. The two-dimensionality, however, also introduces peculiarities: as there are no neighboring atomic planes inhibiting out-of-plane deformations, the presence of dislocations with their associated strain fields may lead to strong out-of-plane corrugations. This can be readily illustrated by considering a plain sheet of paper: try to compress it in the in-plane direction or perhaps pinch it in the center, and it will most certainly not get smaller, but will rather buckle. The importance of three-dimensional (3D) buckling in strained 2D materials has been pointed out earlier [10] , [11] , [12] , [13] , [14] , [15] , [16] . However, as accounting for 3D out-of-plane deformations significantly complicates calculations [12] , such deformations have either been omitted in theoretical studies, or the studied systems have been too small to describe the long-range corrugations [9] , [17] , [18] , [19] , [20] , [21] , [22] , [23] . In order to follow the whole life cycle of a dislocation atom-by-atom, we have here employed AC-HRTEM using the electron beam both to image the dynamics of atoms in a suspended single-layer graphene sheet and to stimulate atomic-level structural changes. It is well known that in graphene, high-energy electron irradiation can induce sputtering of carbon atoms and bond rotations (so-called Stone–Wales transformations) [24] . In our experiment, we used an operating voltage of 80 kV, which is below the static sputtering threshold in graphene. However, thermal vibrations lead to non-zero displacement cross-section and therefore allow occasional sputtering [25] . As the structural changes were of specific interest in our experiment, we increased the temporal frequency of the transformation events by working at exceptionally high beam currents (up to 1 × 10 8 e nm −2 s −1 , that is, one to two orders of magnitude higher than what is typically used for purely structural investigations). The whole life cycle of an edge dislocation is presented below at atomic resolution, including its creation, motion, interaction with other dislocations and eventual annihilation. The dislocations are first formed by sputtering carbon atoms by the energetic electrons, followed by reorganization of the vacancy agglomerates. The dislocations are seen to migrate either via bond rotations or further sputtering of atoms. A markedly long-ranging interaction of the dislocations is observed, and is determined to be mediated by strong out-of-plane buckling of graphene, rather than in-plane strain as assumed previously. Owing to an attractive force acting between the dislocation cores, the cores are driven towards each other, ultimately resulting in the annihilation of the defects. As a whole, these observations comprise the first atomic-scale observation of the full life cycle of dislocations in any material. Birth of dislocations in graphene When carbon atoms are knocked out from the graphene lattice, vacancy-type defects, such as that shown in Fig. 1a are formed. Prolonged irradiation leads to further carbon sputtering, and isolated vacancies agglomerate into larger vacancy structures (see Fig. 1b–d ). It has been predicted that for >10 missing atoms it is energetically favorable for the vacancy agglomerate to locally reorganize into a dislocation dipole terminated by two edge dislocations [19] . This is exactly what can be observed in Fig. 1e , where the vacancies are rearranged into a missing row of atoms in-between the two dislocation cores (see Supplementary Figure S2 for details of the structure). In the following, such dislocations are termed to be pointing away from each other, and dislocations in the opposite orientation are termed to be pointing towards each other. In general, dislocations are created through variations of such a process in our experiment, with a multi-vacancy complex preceding the birth of a dislocation dipole. 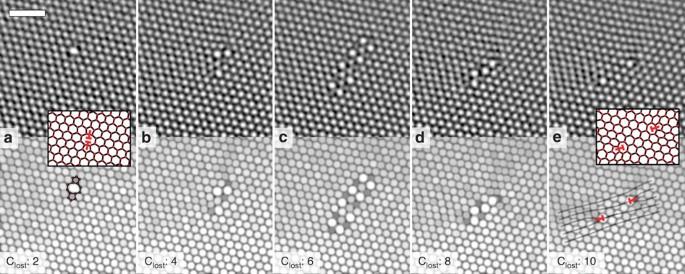Figure 1: The birth of a dislocation dipole in graphene. Two edge dislocations are created via sputtering of carbon atoms and reorganization of the multi-vacancy structure. The upper panels show the original AC-HRTEM images with low-pass Fourier filtering applied and the lower panels show the same frames with maximum filtering applied for better visibility (seeSupplementary Figure S1for details). In panela, two atoms have been removed, forming a divacancy. In each subsequent panelb–etwo more atoms have been removed and the defect has undergone considerable reorganization. In panele, with ten missing atoms, the defect structure has reorganized into a dislocation dipole with two edge dislocations at its ends pointing away from each other. This birth event is shown inSupplementary Movie 1. The scale bar is 1 nm. Figure 1: The birth of a dislocation dipole in graphene. Two edge dislocations are created via sputtering of carbon atoms and reorganization of the multi-vacancy structure. The upper panels show the original AC-HRTEM images with low-pass Fourier filtering applied and the lower panels show the same frames with maximum filtering applied for better visibility (see Supplementary Figure S1 for details). In panel a , two atoms have been removed, forming a divacancy. In each subsequent panel b – e two more atoms have been removed and the defect has undergone considerable reorganization. In panel e , with ten missing atoms, the defect structure has reorganized into a dislocation dipole with two edge dislocations at its ends pointing away from each other. This birth event is shown in Supplementary Movie 1 . The scale bar is 1 nm. Full size image Motion of dislocations Edge dislocations can migrate in the graphene lattice by climbing and gliding in different directions as schematically shown in Fig. 2 . In the climb motion, atoms are either added or removed next to the dislocation core (see Supplementary Figure S3 for details). In practice, under our experimental conditions, removal of atoms happens frequently, while adding new atoms into the lattice is a more rare event. Nevertheless, filling of a divacancy was also observed in our experiment (see Supplementary Figure S4 ). This leads to climb happening predominantly in the direction shown in the figure (the atoms marked with crosses are removed). We would like to point out that atoms next to the dislocation core are much more frequently sputtered in our experiment, as compared to the intact parts of the lattice. This indicates a lowered displacement threshold for those atoms, which was also validated by our simulations (see Supplementary Figure S5 ). Simple glide motion is facilitated by a Stone–Wales transformation, where two neighboring carbon atoms (marked with the ellipse in the figure) rotate by 90° around their midpoint, resulting in the movement of the dislocation by 0.25 nm (see Supplementary Figure S6 for details). HRTEM images of these steps are shown in Fig. 2b–e , and have been also presented by Warner et al . 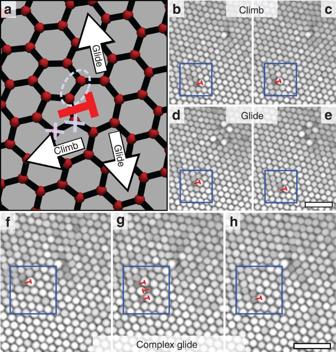Figure 2: Migration of dislocations in graphene. In panela, the possible directions of movement are presented schematically. A climb step of one lattice plane requires removal of two carbon atoms (marked with crosses). Climb in the opposite direction is in principle possible via introduction of extra carbon atoms, but this is not observed in our experiment. A simple glide step requires rotation of a pair of carbon atoms (marked with the ellipse) by 90° around their middle point. Here, the number of atoms remains the same. The maximum filtered AC-HRTEM images in panelsbandcshow the basic climb step in action. Panelsdandeshow a glide step. Panelsftohshow a more complex glide step, where first a bond rotation takes place next to the dislocation core, and a subsequent rotation of another bond brings the dislocation two steps downwards. Even more complex migration process can be observed underway at the top right corners of panelsdandeand inSupplementary Movie 2. The scale bars are 1 nm. [9] Figure 2: Migration of dislocations in graphene. In panel a , the possible directions of movement are presented schematically. A climb step of one lattice plane requires removal of two carbon atoms (marked with crosses). Climb in the opposite direction is in principle possible via introduction of extra carbon atoms, but this is not observed in our experiment. A simple glide step requires rotation of a pair of carbon atoms (marked with the ellipse) by 90° around their middle point. Here, the number of atoms remains the same. The maximum filtered AC-HRTEM images in panels b and c show the basic climb step in action. Panels d and e show a glide step. Panels f to h show a more complex glide step, where first a bond rotation takes place next to the dislocation core, and a subsequent rotation of another bond brings the dislocation two steps downwards. Even more complex migration process can be observed underway at the top right corners of panels d and e and in Supplementary Movie 2 . The scale bars are 1 nm. Full size image These basic climb and glide steps are not necessarily typical for the dislocations, however, as migration tends to take more complex forms, such as that displayed in Fig. 2f–h . Here, the dislocation first transforms via a bond rotation into a chain of dislocations (dubbed a ‘dislocation worm’ elsewhere [13] ), which has earlier been predicted to have a lower formation energy under strained conditions. Subsequently, another bond rotation moves the dislocation two glide steps (0.5 nm) away from the original site. Even more complex migration processes can be seen underway in the upper right corners of Fig. 2d and e and in Supplementary Movie 2 . Interaction of dislocations In order to predict the effect of the removal of the string of atoms on the structure of graphene, we conducted conjugate gradient structural relaxations of a large graphene supercell (~25 × 25 nm and ~24,000 atoms) containing a dislocation dipole in various configurations, employing an analytical force field [26] to describe the C–C interactions. The missing string of atoms induces tensile strain in-between the dislocation cores and compression outside this area [11] . However, as the stress required to stretch the surrounding exceedingly large graphene sheet is very small and the compressional strain can be released via out-of-plane corrugations (the energy constants characterizing in-plane and flexural stiffness differ by two orders of magnitude [27] ), the width of the system was set to such a value that strain across the dislocation dipole is zero and the graphene sheet was allowed to buckle. Counter-intuitively, the damaged parts where the atoms were removed stay close to the pristine state, whereas the rest of the sheet is buckled, with slowly fading out-of-plane deformations extending over large distances. However, if the corrugations of two dislocation cores pointing towards each other (that is, originating from different dipoles) overlap, they can terminate each other. Examples of such situations are depicted in Fig. 3c and d . 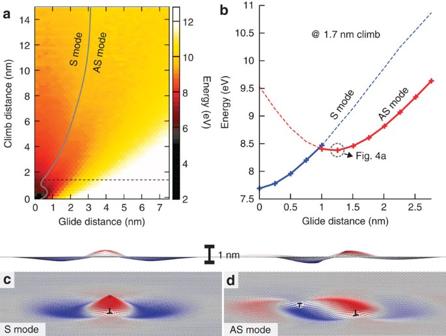Figure 3: 3D buckling and interaction of dislocations pointing towards each other. Panelashows the potential energy of the system depending on the relative orientation of the dislocations in terms of glide and climb distance. Panelbshows the energies of the two different buckling modes as a function of glide distance at a fixed climb distance of 1.7 nm. Panelscanddvisualize different buckling modes, which depend on whether the dislocations extend out of the plane symmetrically (S mode) or anti-symmetrically (AS mode). Red color indicates elevation and blue depression in the positions of the carbon atoms. On the left side of the solid line in panelathe S mode is energetically favorable, and the AS mode is favorable to the right of the line. The horizontal dotted line indicates the climb distance corresponding to the data presented in panelb. Figure 3: 3D buckling and interaction of dislocations pointing towards each other. Panel a shows the potential energy of the system depending on the relative orientation of the dislocations in terms of glide and climb distance. Panel b shows the energies of the two different buckling modes as a function of glide distance at a fixed climb distance of 1.7 nm. Panels c and d visualize different buckling modes, which depend on whether the dislocations extend out of the plane symmetrically (S mode) or anti-symmetrically (AS mode). Red color indicates elevation and blue depression in the positions of the carbon atoms. On the left side of the solid line in panel a the S mode is energetically favorable, and the AS mode is favorable to the right of the line. The horizontal dotted line indicates the climb distance corresponding to the data presented in panel b . Full size image To study how this affects the energetics of the system, the potential energy of the system was mapped as a function of glide and climb distance of the cores. The resulting energy landscape is shown in Fig. 3a , with each point normalized to the number of atoms. Towards the lower left corner, the dislocations come closer to each other. Going up in the map means increasing the climb distance and the number of atoms, whereas going right increases the glide distance. As bond rotations happen much more frequently than sputtering, dislocations can easily migrate towards an energy minimum in the horizontal direction for any given vertical climb distance. The general trend in the energy map is clear: the closer the dislocations come, the lower the energy becomes, resulting in attractive force acting between the dislocations over large distances. The cores now effectively form a dislocation dipole with a row of extra atoms in-between them. The buckling can take place in different modes, depending on whether the individual dislocations are extended out of the plane in the same or opposite directions. These modes are presented in Fig. 3c and d , where the symmetrical extension is named the S mode, and anti-symmetrical one the AS mode. The energetics change depending on which mode is taking place, which can be seen in Fig. 3b , where the energy is plotted at a fixed climb distance of 1.7 nm. The system finds its global energy minimum in the S mode at zero glide distance, and the energy in this mode increases monotonously with increasing glide distance. The AS mode has significantly higher energy at small glide distances, but as the distance increases, the energy goes down, and the mode becomes energetically favorable after a certain crossing point, the location of which depends on the climb distance. The AS mode has an energy minimum at a location that depends on the climb distance (1.2 nm for the presented case), after which the energy starts to increase, leading to an attractive force also in this mode. As is shown later, in the experiment, the dislocations tend to reside exactly at the distance where the energy minimum is predicted to be. The calculated significant out-of-plane buckling was confirmed by our experiments. Traditionally, TEM is considered to be insensitive to 3D features of a sample, due to the inherently wide depth of focus of the instrument. However, in an AC-HRTEM image, the brightness of the center of a carbon polygon is sensitive to its projected size. This means that if a polygon is tilted, for example, due to a corrugation, its center becomes less bright. Compared to the lattice contrast, these variations are small, and hence they are not clearly visible without image processing (see Fig. 4a ). However, by applying maximum filtering on the digital images, where the brightest pixels are expanded to cover their neighborhood up to a predefined radius, the variations in the polygon brightnesses can be amplified (see Supplementary Figure S1 for details). Similar information can be extracted using geometrical phase analysis, as was demonstrated recently by Ortolani et al . [28] . However, the interpretation of geometrical phase analysis results is biased towards reading the apparent reduction in bond lengths as compression rather than tilting, as in a previous study [9] , where as high as 27% compression of bonds was reported next to the dislocation cores. 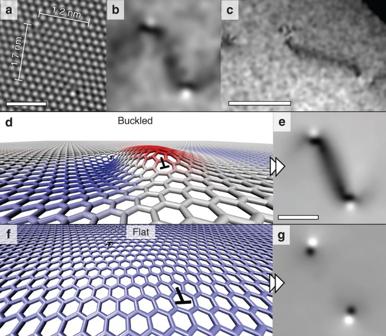Figure 4: Observing the 3D buckling under the electron microscope. In panela, a dislocation dipole imaged using HR-TEM is shown. The glide and climb distances coincide with the local energy minimum in the energy graph ofFigure 3c. In panelbthe same image is shown after extensive image filtering (seeSupplementary Figure S1for details). A dark contrast line becomes visible, connecting the dislocation cores. Panelcshows a larger field-of-view image with corrugations extending over a long distance (seeSupplementary Figure S7andSupplementary Movie 3for more examples). Paneldshows a perspective-view of a graphene sheet relaxed in a computer simulation, with a dislocation dipole with the same configuration as seen in panela. Paneleshows a simulated and filtered AC-HRTEM image of the structure in paneld. Panelfshows the same dislocation configuration, but relaxed with the system constrained to be flat, and panelgshows a simulated and filtered AC-HRTEM image of this structure. The scale bars are 1 nm inaande, and 5 nm inc. Figure 4: Observing the 3D buckling under the electron microscope. In panel a , a dislocation dipole imaged using HR-TEM is shown. The glide and climb distances coincide with the local energy minimum in the energy graph of Figure 3c . In panel b the same image is shown after extensive image filtering (see Supplementary Figure S1 for details). A dark contrast line becomes visible, connecting the dislocation cores. Panel c shows a larger field-of-view image with corrugations extending over a long distance (see Supplementary Figure S7 and Supplementary Movie 3 for more examples). Panel d shows a perspective-view of a graphene sheet relaxed in a computer simulation, with a dislocation dipole with the same configuration as seen in panel a . Panel e shows a simulated and filtered AC-HRTEM image of the structure in panel d . Panel f shows the same dislocation configuration, but relaxed with the system constrained to be flat, and panel g shows a simulated and filtered AC-HRTEM image of this structure. The scale bars are 1 nm in a and e , and 5 nm in c . Full size image Figure 4a shows an AC-HRTEM micrograph of two interacting dislocation cores. Panel b presents the same image after processing. A clearly visible dark ridge connecting the dislocation cores is observable, indicating a reduced projected size of the polygons along that line. This can be attributed either to corrugations or compressive strain, as both of them reduce the projected size of the polygons. To identify which scenario takes place in the experiment, the same dislocation configuration was relaxed first by allowing the structure to buckle and next by constraining the geometry to be flat. The first relaxation resulted in the corrugated structure visualized in Fig. 4d . The structure was subsequently used for HR-TEM image simulation. Applying identical filtering as was used for the experimental image resulted in strikingly similar features as compared with the experiment. The total energy of the flat relaxed system is 17 eV higher than in the previous buckled case. Further on, its simulated and filtered image ( Fig. 4g ) proved to be in disagreement with the experimental one. Most importantly, the dark ridge connecting the dislocations is absent. Similar simulated image to Fig. 4e would result from a flat atomic structure with the same in-plane coordinates as in the buckcled structure. The total energy of such a configuration ends up 145 eV higher in our simulation, however. Thus, the contrast observed in the experimental image is likely due to out-of-plane buckling of the graphene sheet rather than bond contraction, and the corrugations in the experiment follow the prediction of the simulations. The markedly long-range nature of the corrugation-mediated interactions of dislocations and other defects can be observed in Fig. 4c . The dark ridge extends over the length of 7 nm terminating at separate defects. More examples with even longer ranges are presented in Supplementary Figure S7 and Supplementary Movie 3 . One can further conclude that even at fairly low concentrations, point defects in graphene can no longer be considered isolated. Instead they form an interconnected network, as the strain fields or ‘corrugation fields’ of interacting defects strongly affect the energetics of the system. Annihilation of dislocations As edge dislocations in graphene pointing towards each other have net attraction, and both the glide and climb mechanisms are activated by the electron beam, dislocations should migrate towards each other and undergo annihilation. This is precisely what we observed experimentally. In Fig. 5a , four dislocations are present. The dark ridges, indicating the interlocking of the corrugations of the dislocations, are visible in the filtered images. The left-most dislocations approach each other, following the previously predicted path of local energy minima. Finally, they disappear, leaving a perfect hexagonal graphene lattice behind. At close proximity, a larger reorganization takes place (panel d). This reconstruction resembles the intermediate configurations in Fig. 1 , but actually has extra atoms instead of vacancies, consisting of two adatom pairs and a Stone–Wales defect. 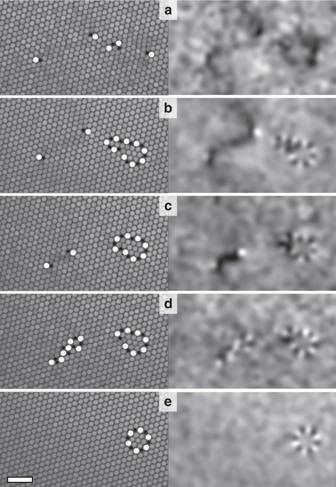Figure 5: Attraction and annihilation of dislocations in graphene. Panelahas four dislocations. The two left-most dislocations interact through the AS mode and the right-most through S mode. In the subsequent panelsbandcthe left-most dislocations migrate towards each other, making a more complex rearrangement in paneldbefore undergoing annihilation (panele), leaving behind defect-free graphene. The right-most dislocations cause a reorganization of the lattice along the connecting corrugation, resulting in a closed grain boundary loop (also called the flower defect). The dislocations themselves disappear, and the density of the sheet returns to the pristine value, but the grain boundary loop is left behind. Here, white and black circles are overlaid on the pentagons and heptagons to further improve the visibility of the structures. The scale bar is 1 nm. Figure 5: Attraction and annihilation of dislocations in graphene. Panel a has four dislocations. The two left-most dislocations interact through the AS mode and the right-most through S mode. In the subsequent panels b and c the left-most dislocations migrate towards each other, making a more complex rearrangement in panel d before undergoing annihilation (panel e ), leaving behind defect-free graphene. The right-most dislocations cause a reorganization of the lattice along the connecting corrugation, resulting in a closed grain boundary loop (also called the flower defect). The dislocations themselves disappear, and the density of the sheet returns to the pristine value, but the grain boundary loop is left behind. Here, white and black circles are overlaid on the pentagons and heptagons to further improve the visibility of the structures. The scale bar is 1 nm. Full size image The right-most dislocation pair also causes reorganization of the lattice in-between them. In this case, however, the reorganization leads to the formation of a small closed grain boundary loop (the flower defect). They have been reported to form under an electron beam [29] and have been demonstrated to be highly stable [30] . While the dislocations undergo annihilation and the atomic density becomes equal to the pristine lattice, the small grain is left behind. This sequence can be seen in Supplementary Movie 4 . To the best of our knowledge, these are the first direct atomic-scale observations of the annihilation process of edge dislocations. The more traditional way, however, for a dislocation to be removed from a crystal is the migration of the core to the edge of the crystal. Corresponding examples are presented in Supplementary Movies 5 and 6 . The whole life cycle of an edge dislocation in graphene, including its creation, motion, interaction with other dislocations, and finally annihilation was presented—atom-by-atom and step-by-step—using an aberration-corrected high-resolution electron microscope for both imaging and inducing transformations in the atomic structure. The dislocations were created by sputtering carbon atoms due to impacts of energetic electrons, and subsequent reorganization of the graphene lattice. The dislocations were seen to migrate through the bond rotation-mediated glide mechanism, as well as the climb mechanism facilitated by removal of carbon atoms. A markedly long-ranging interaction of the dislocations was observed. The interaction is driven by strong out-of-plane buckling of graphene, instead of the previously assumed in-plane strain, as corroborated by atomistic computer simulations, as well as image-filtering techniques applied to the experimental micrographs. An attractive force acting between dislocation cores was seen to drive the cores towards each other, ultimately resulting in the annihilation of the defects, leaving behind defect-free graphene. To our knowledge, this is the first atomic-scale observation of the full life cycle of a dislocation—a concept of pivotal importance in materials science. Experimental HR-TEM experiments were carried out in a Cs-corrected FEI Titan 80–300 microscope at an operation voltage of 80 kV. In order to reduce the energy spread of the electron beam, the extraction voltage of the field emission source was reduced to 2 kV. The spherical aberration was set to 2 μm, and images were recorded at Scherzer defocus. Under these conditions, atoms appear dark. By strongly converging the beam it is possible to obtain beam current densities up to 1 × 10 8 e nm −2 s −1 as measured via the known conversion rate of the CCD camera. Of course under these conditions, the illumination is very inhomogeneous (intensity in the center is about a factor of two higher than in the edges). Continuous imaging was possible by working at the highest microscope magnification and reducing the exposure time of the Gatan Ultrascan XP CCD camera to 0.2 s at binning 2 (readout time 0.6 s). For the acquisition we used a post-specimen blanker. In consequence, the dose on the sample was approximately four-times higher than the dose on the CCD. The recording was continued until a large hole formed in the sample (see Supplementary Figure S8 and Supplementary Movies 7 and 8 ). The resulting image sequences were background-subtracted and drift-compensated. For better visibility of the defect structures, additional filtering turned out to be very helpful as explained in Supplementary Figure S1 . Computational The atomic structure of graphene with dislocations was studied by carrying out structural relaxations of a graphene sheet with a size of ~25 × 25 nm and consisting of ~24,000 carbon atoms, exact number depending on the dislocation separation. The interatomic forces were described by an analytical bond-order potential [26] . In the calculations, always two oppositely oriented dislocation cores were placed with different glide and climb distances, and the resulting structures were relaxed using the conjugate gradient algorithm as implemented in the in-house code Relaxat. Similar approach has earlier been applied to modeling strained carbon systems [13] , [15] . In the displacement threshold calculation the interatomic forces were described via the density functional-based tight binding formalism [31] . In these molecular dynamic simulations, the atom of interest was assigned momentum in the normal direction relative to the graphene sheet and after the simulation time of 300 fs, it was determined whether the atom was detached from rest of the structure. A binary search algorith was used to pinpoint the threshold energy. The simulated system consisted of 152 carbon atoms, with two dislocations separated by five climb steps at zero glide distance. A single k-point was used for the calculations and the simulation was run at 0 K. The HR-TEM image simulations were conducted using the QSTEM software using the multislice algorithm [32] . In the simulations, spherical aberration coefficient of 2 μm, focal spread of 7 nm and Scherzer focus were used. How to cite this article: Lehtinen, O. et al . Atomic scale study of the life cycle of a dislocation in graphene from birth to annihilation. Nat. Commun. 4:2098 doi: 10.1038/ncomms3098 (2013).